Binding of herpes simplex virus glycoprotein D to nectin-1 exploits host cell adhesion Multiple surface envelope proteins are involved in the human herpes simplex virus type 1 entry and fusion. Among them, glycoprotein D (gD) has an important role by binding to the host receptors such as herpes virus entry mediator and nectin-1. Although the complex structure of gD with herpes virus entry mediator has been established, the binding mode of gD with the nectin-1 is elusive. Nectin-1 is a member of the immunoglobulin (Ig)-like (three Ig-like domains) cell adhesion molecules and is believed to form a homodimer to exert its functions. Here we report the complex structure of gD and nectin-1 (three Ig domains), revealing that gD binds the first Ig domain of nectin-1 in a similar mode to the nectin-1 homodimer interaction. The key amino acids responsible for nectin-1 dimerization are also used for gD/nectin-1 binding. This result indicates that binding of gD to nectin-1 would preclude the nectin-1 dimerization, consequently abolishing its cell adhesion function. Herpesvirus infections are widely spread throughout the world population. The virus is believed to be a major cause of human viral diseases, second only to influenza and common cold viruses. The diseases caused by herpes virus infection can be overt or silent for many years, and an infection in humans usually results in an individual being a life-long virus carrier. Though the disease usually is mild, it can be severe and life-threatening in immunocompromised patients [1] . Therefore, understanding of the molecular pathogenesis of the virus infection is of interest for disease control and prevention. Herpesvirus is a group of enveloped viruses, forming Family Herpesviridae with subdivision into three subfamilies. Herpes simplex virus (HSV) belongs to the α-herpesvirus subfamily. There are two main types of HSV, HSV-1 and HSV-2, which infect humans. HSV-2 mainly causes genital lesions, whereas HSV-1 is involved in both oral and genital infections [1] , [2] . In the latent stage of infection, the virus resides in neurons of sensory ganglia [3] . The initial infection of HSV-1 or HSV-2 starts with virus entry into host cells. Despite a remaining controversy in the literature as to whether virus enters by fusion alone or both fusion and endocytosis, it is widely accepted that HSV entry is mainly through attachment and fusion, a multi-event that is mediated by interaction of viral envelope protein/s with host surface receptor/s [4] , [5] . There are 11 enveloped proteins on the virus surface of HSV-1 and it is believed that at least 5 of them (gC, gB, gD, gH and gL) are involved in this process [4] , [6] . Glycoprotein C and B (gC, gB) could tether viruses onto host cell surface by interacting with heparin sulphate proteoglycan (HSPG), thereby initializing the virus attachment [7] , [8] . On the other hand, gB, for which several ligands other than HSPG, are reported recently including PILRα and NMHC-IIA, mediates membrane fusion by forming a core fusion machinery with gH/gL [9] , [10] , [11] , [12] . The glycoprotein gD is believed to trigger a cascade of events activating fusion process via binding to receptors [13] , [14] . The gC/HSPG interaction is important yet non-essential in HSV entry [8] , gD/receptor interaction is the key to trigger fusion and is considered an essential step before interactions between gB and gH/gL [11] . There are at least three cellular receptors for gD, namely herpes virus entry mediator (HVEM), nectin-1 and 3- O -sulfonated derivatives of heparin sulphate [15] . Elucidation of the molecular basis of the interaction between gD and its cellular receptors is important for our understanding of virus entry and drug design. Although the structural basis of gD binding to HVEM has been resolved [16] , the complex structures of gD with the other two receptors remain elusive. Nectin-1 is a member of the nectin and nectin-like (Necl) molecules family, which consist of nine members (nectin 1–4 and Necl 1–5) [17] . This family of the molecules belongs to immunoglobulin (Ig)-like cell adhesion molecules (CAMs) and has important roles in mediation of cell–cell adhesion and some other regulatory functions including cell polarization, differentiation, movement, proliferation, survival and immune regulation [18] , [19] . Homophilic or heterophilic dimerization is believed to be important in facilitating the function of the members of this family [17] . Nectin-1 has been illustrated to form either homodimers (believed to form both cis - and trans -dimers) or heterodimers with other family members (for example, with nectin-3, nectin-4 and Necl 1) in its cell–cell adhesion [20] . From the elucidation of the cis -homodimer structure it has been proposed that the cis -homodimer of nectin-1 binds to HSV-1 gD [21] . However, previous functional data are controversial in regards to the binding mode of nectin-1 with gD [21] , [22] , although it has been unambiguously demonstrated that the soluble ectodomain of gD indeed inhibited the nectin-1-mediated cell–cell adhesion [23] , [24] . The crystal structure of the gD ectodomain shows it has an Ig-like fold core (V-set Ig) that is flanked by large N- and C-terminal extensions. The core Ig-like domain is closely related to immune cell co-stimulatory molecules, such as CD2, CD28 and CD80 (ref. 16 ). The structure of the complex between gD and HVEM shows that the N-terminal hairpin extension dominates the binding and that the extension undergoes some conformational changes upon receptor binding [16] . Nectin-1 has three Ig-like domains in its ectodomain, the first is a V-set Ig, whereas the second and the third are C-set Igs. A recent crystal structure of the three Ig-like domains of nectin-1 shows it forms a homodimer through the first Ig domain [21] . Here, to further establish the molecular basis of HSV fusion to the host cell, we solve the crystal structure of the gD/nectin-1 complex and the results surprisingly show that the binding interface of gD to nectin-1 is very similar to that of the nectin-1 homodimer interface. The binding chemical stoichimetry is 1:1 (gD:nectin-1); consequently, this binding mode abolishes the nectin-1 dimerization and therefore makes nectin-1 mediated cell–cell adhesion impossible. A 1:1 binding mode of the gD/nectin-1 complex The primary focus of this study was to resolve the atomic structure of HSV-1 gD bound to nectin-1. In terms of a previous report showing that a gD truncation at residue 285 (gD285) exhibits much higher affinity for nectin-1 than the longer ectodomain gD molecule (residues 1–306), gD285 protein was prepared for co-crystallization trials [13] , [25] . With a 3-M excess of the gD protein to the three-Ig nectin-1 protein, a complex crystal was successfully obtained which could diffract to 3.2 Å The structure was solved using the molecular replacement method, and finally refined to R work =0.321 and R free =0.344, respectively, (for details, see Methods ). Despite limited resolution, which prevents an in-depth insight into the details of gD/nectin-1 interaction, the structure was, to our knowledge, the first one to establish the direct binding mode of the gD/nectin-1. 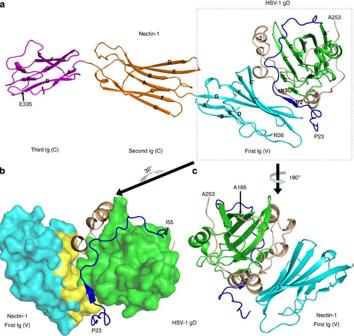Figure 1: Overall structure of the gD/nectin-1 complex. (a) A ribbon representation of the gD/nectin-1 complex structure. HSV-1 gD is coloured green and labelled according to Carfiet al.16. The N- and C-terminal extensions within gD, which contains nectin-1 binding site, are highlighted in blue and gold, respectively. The three-domained nectin-1 was labelled as in a recent report by Naritaet al.21The first V-set Ig domain (first Ig) of nectin-1 is coloured cyan. The second (second Ig) and the third (third Ig) domains, both exhibiting a C-set Ig fold, are coloured orange and magenta, respectively. Clearly, only the first Ig V-set domain of nectin-1 binds gD. (b,c) A magnified view of the gD molecule and the nectin-1 first Ig domain within the complex structure. The V-set Ig core of gD and the first Ig domain of nectin-1 are also shown in a surface representation in (b) to highlight the N- and C-terminal extensions in gD (including the nectin-1 contact residues). The residues bordering these terminal extensions (P23, I55, A185 and A253) are indicated and labelled. The interactive surface in Ig-like V-set domain of nectin-1 is coloured yellow in (b). The dash-line boxed part in (a) is clockwise rotated for about 30° or horizontally flipped for about 180° to yield (b) and (c), respectively. As shown in Figure 1a , in the complex structure, only one gD molecule and one nectin-1 molecule existed per asymmetric unit. Electron densities could be observed for amino acids P23-A253 of gD protein, with terminal residues 1–22 and 254–285 being invisible due to disorder. Overall, HSV-1 gD adopts a similar fold as previously reported [16] . Nine strands (A′, B, C, C′, C″, D, E, F and G) are arranged in an Ig-like V-set domain manner to form a β-barrel core (V-set Ig, residues 56–184). This compact core is further wrapped by the surface components including four α-helices (α1, α1′, α2 and α3), two short strands (Str2 and Str3) and abundant loops, most of which belong to the N-terminal (residues P23 to I55) and C-terminal (residues A185 to A253) extensions. The nectin-1 binding site of HSV-1 gD (4.5 Å cutoff) mainly locates in these terminal extensions ( Fig. 1b,c ). Figure 1: Overall structure of the gD/nectin-1 complex. ( a ) A ribbon representation of the gD/nectin-1 complex structure. HSV-1 gD is coloured green and labelled according to Carfi et al . [16] . The N- and C-terminal extensions within gD, which contains nectin-1 binding site, are highlighted in blue and gold, respectively. The three-domained nectin-1 was labelled as in a recent report by Narita et al . [21] The first V-set Ig domain (first Ig) of nectin-1 is coloured cyan. The second (second Ig) and the third (third Ig) domains, both exhibiting a C-set Ig fold, are coloured orange and magenta, respectively. Clearly, only the first Ig V-set domain of nectin-1 binds gD. ( b , c ) A magnified view of the gD molecule and the nectin-1 first Ig domain within the complex structure. The V-set Ig core of gD and the first Ig domain of nectin-1 are also shown in a surface representation in ( b ) to highlight the N- and C-terminal extensions in gD (including the nectin-1 contact residues). The residues bordering these terminal extensions (P23, I55, A185 and A253) are indicated and labelled. The interactive surface in Ig-like V-set domain of nectin-1 is coloured yellow in ( b ). The dash-line boxed part in ( a ) is clockwise rotated for about 30° or horizontally flipped for about 180° to yield ( b ) and ( c ), respectively. Full size image On the other hand, for the nectin-1 molecule within the complex structure 300 amino acids were visible in the electron density map, extending from N36 to E335 ( Fig. 1a ). This three-Ig domain protein retains its rod shape as observed in a recent cis -dimer structure [21] . The first domain (first Ig) of nectin-1 is composed of nine strands (A, B, C, C′, C″, D, E, F and G), forming a typical Ig-like V-set fold. Both the second (second Ig) and the third (third Ig) domains contain only seven anti-parallel β-strands (A–G), and are thereby classified as the C-set Ig-like domains. On the whole, the nectin-1 molecule interacts extensively with HSV-1 gD only through its first Ig domain ( Fig. 1b,c ), which is largely consistent with previous results of mutational and in-vitro binding assays [25] , [26] , [27] . Further analysis of the complex structure unexpectedly reveals that the interaction interface between gD and nectin-1 is the same as that mediating cis -dimerization of the two nectin-1 molecules [21] . This unique interaction mode, together with the observation of only one gD molecule and one nectin-1 molecule per asymmetric unit within the crystal, strongly supports a 1:1 (1 gD monomer with 1 nectin-1 monomer) binding mode for the gD/nectin-1 complex. Nectin-1 is a monomer–dimer equilibrium and monomer binds gD We next set out to compare the three protein species (nectin-1 alone, gD alone and the gD/nectin-1 complex) by analytical size-exclusion chromatography using a calibrated Superdex 200 10/300 GL column (GE Healthcare). 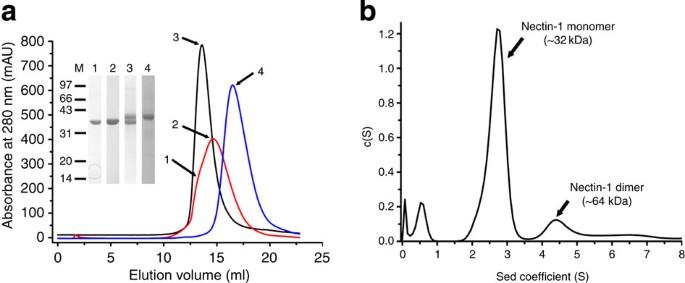Figure 2: Biochemical and biophysical characterization of the prepared proteins. (a) Size-exclusion analysis of nectin-1 (red), gD (blue) and the gD/nectin-1 complex (black). The chromatographs of the three prepared protein species on a calibrated Superdex 200 column (10/300 GL), as well as the separation profiles of each pooled samples (peaks 1, 2, 3 and 4) on SDS–PAGE, are shown. Clearly shown are that peak 3 has two proteins, gD and nectin-1; the shoulder peak, peak 1, has nectin-1 (dimer); and peak 2 has nectin-1 as well (monomer); peak 4 is gD. (b) The analytical ultracentrifugation profile of nectin-1 shows the sedimentation coefficient distribution analysis c(s). The two identified species, whose corresponding MWs were calculated to be 32 and 64 kDa, respectively, are indicated, demonstrating the monomer–dimer equilibrium for nectin-1 in solution. As shown in Figure 2a , the gD protein eluted as a single peak at 16 ml, corresponding to an apparent molecular weight (M W ) of 36 kDa. This is consistent with the previous reports showing that the ectodomain of gD exists as a monomer in solution [13] , [16] , whereas the complex of gD with nectin-1 resulted a shift of about 2 ml in elution volume to about 14 ml, with the M W calculated to be 70 kDa. This protein species is in a good accordance with the M W of one gD molecule in combination with a single nectin-1, which in turn further supports the 1:1 binding mode as observed in the complex structure. Figure 2: Biochemical and biophysical characterization of the prepared proteins. ( a ) Size-exclusion analysis of nectin-1 (red), gD (blue) and the gD/nectin-1 complex (black). The chromatographs of the three prepared protein species on a calibrated Superdex 200 column (10/300 GL), as well as the separation profiles of each pooled samples (peaks 1, 2, 3 and 4) on SDS–PAGE, are shown. Clearly shown are that peak 3 has two proteins, gD and nectin-1; the shoulder peak, peak 1, has nectin-1 (dimer); and peak 2 has nectin-1 as well (monomer); peak 4 is gD. ( b ) The analytical ultracentrifugation profile of nectin-1 shows the sedimentation coefficient distribution analysis c(s). The two identified species, whose corresponding M W s were calculated to be 32 and 64 kDa, respectively, are indicated, demonstrating the monomer–dimer equilibrium for nectin-1 in solution. Full size image Results from size-exclusion chromatography using a Superdex 200 column showed nectin-1 to elute with a main peak at 15 ml combined with a shoulder at 14.5 ml, indicating the presence of two species, corresponding to dimer and monomer in solution ( Fig. 2a ). The pooled protein sample of peak 2 was then subjected to ultracentrifugation sedimentation analysis. As shown in Figure 2b , the equilibrium data reveals two protein species with M W of about 32 and 64 kDa, respectively, demonstrating the presence of both monomeric and dimeric nectin-1 in solution. It is also noteworthy that the amount of nectin-1 dimer was calculated to be only about 11% of that of monomer, indicating that at lower concentrations, nectin-1 predominantly existed as a solvent monomer. Therefore, taken together, these analyses confirm the monomer–dimer equilibrium of nectin-1 in solution. Despite great efforts carried out to try and obtain the gD/nectin-1 complex crystals, the only successful attempts were those in which the purified monomeric nectin-1 was used for co-crystallization with 3-M excess of soluble gD. Nevertheless, with the dimeric nectin-1, the yielded crystals were invariably nectin-1 molecule alone, which could be interpreted as further supportive evidence for the 1:1 binding mode. The intimate interaction between HSV-1 gD and nectin-1 has been observed both in vitro and in vivo [22] , [28] . In several previous studies using eukaryotic cell expressed gD and nectin-1, the binding affinity of the two proteins has been demonstrated to be in the two-digit nanomolar range (38–70 nM) [13] , [25] , [29] . In this study, with immobilized Escherichia coli -expressed/refolded nectin-1, surface plasmon resonance (SPR) analysis using BIAcore showed a potent binding capability to soluble HSV-1 gD ( Fig. 3 ). The calculated dissociation constant ( K D ) of gD and nectin-1 was determined to be 17.1 nM, with K on =1.14×10 5 M −1 s −1 and K off =18.9×10 −4 s −1 , respectively. The results indicate that HSV-1 gD binds E. coli -expressed/refolded nectin-1 with a similar affinity to the eukaryotic cell expressed nectin-1. 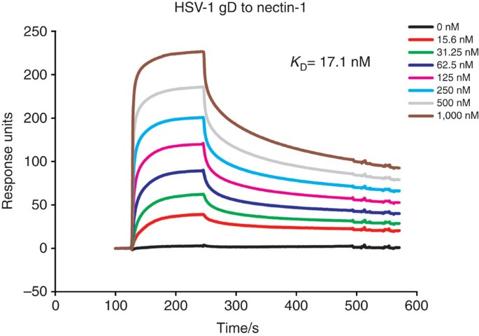Figure 3: Binding affinity of the gD/nectin-1 complex measured using BIAcore method. Gradient concentrations (ranging from 15.6–1000 nM) of HSV-1 gD were injected through flow cells immobilized with nectin-1. The kinetic profiles are shown. The dissociation constant (KD) of the gD/nectin-1 complex was calculated to be 17.1 nM. Figure 3: Binding affinity of the gD/nectin-1 complex measured using BIAcore method. Gradient concentrations (ranging from 15.6–1000 nM) of HSV-1 gD were injected through flow cells immobilized with nectin-1. The kinetic profiles are shown. The dissociation constant ( K D ) of the gD/nectin-1 complex was calculated to be 17.1 nM. Full size image gD binds the same patch as the nectin-1 homodimer interface Despite the limitation of low resolution (3.2 Å) for the gD/nectin-1 complex structure solved here, the interaction interface within the respective contacting molecules could be defined unambiguously. We first scrutinized nectin-1 for those residues that could potentially interact with HSV-1 gD. A total of 22 amino acids were demonstrated to locate within a distance of 4.5 ˚Å from gD ( Table 1 ), thereby could, at least, contact the gD molecule via van der Waals interaction. Of these residues, over half of them were amino acids of hydrophilic (polar or acidic or basic) characters, indicating the important roles that polar contacts should have in the intimate binding of gD to nectin-1. On the whole, all these interface residues reside in the [CC′C″FG] sheet of the V-set first Ig domain of nectin-1, forming an extended contacting patch ( Fig. 4a ). Table 1 Amino acids involved in gD/nectin-1 interaction in comparison with nectin-1 homodimer. 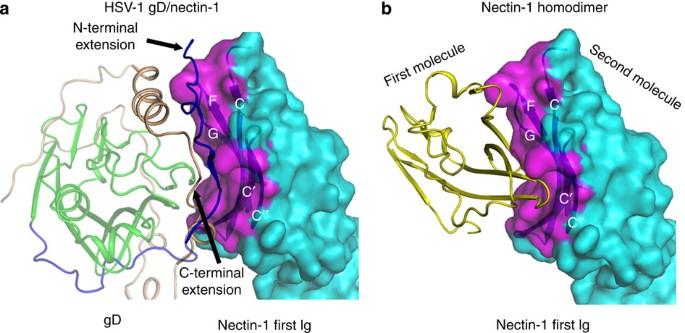Figure 4: Comparison of the binding modes between nectin-1 homo-dimer and gD/nectin-1 heterodimer. The interaction interface within nectin-1 (cyan) contacting gD (Ig core in green, N-terminal extension in blue, C-terminal extension in gold), or contacting the other nectin-1 molecule (yellow) is presented. Nectin-1 is shown in surface representation, with the interface being highlighted by magenta colour. The [CC′C″FG] sheet in which those interface residues reside are presented in a ribbon mode and labelled. The N- and C-terminal extensions in gD are also highlighted. (a) gD/nectin-1 heterodimer. (b) nectin-1 homodimer. gD/nectin-1 heterodimer and nectin-1 homodimer clearly interface via the same nectin-1 region. Full size table Figure 4: Comparison of the binding modes between nectin-1 homo-dimer and gD/nectin-1 heterodimer. The interaction interface within nectin-1 (cyan) contacting gD (Ig core in green, N-terminal extension in blue, C-terminal extension in gold), or contacting the other nectin-1 molecule (yellow) is presented. Nectin-1 is shown in surface representation, with the interface being highlighted by magenta colour. The [CC′C″FG] sheet in which those interface residues reside are presented in a ribbon mode and labelled. The N- and C-terminal extensions in gD are also highlighted. ( a ) gD/nectin-1 heterodimer. ( b ) nectin-1 homodimer. gD/nectin-1 heterodimer and nectin-1 homodimer clearly interface via the same nectin-1 region. Full size image With a recently reported cis -homodimer structure (PDB code: 3ALP) of nectin-1, we investigated the dimerization interface of this adhesion molecule by selection of those residues ≤4.5 Å from the other molecule. Unexpectedly, the same patch as observed in the gD/nectin-1 complex structure was revealed ( Fig. 4b ). Of those 22 amino acid residues mediating nectin-1 dimerization, 19 were also involved in the binding to HSV-1 gD ( Table 1 ). Therefore, nectin-1 uses almost the same interface to interact with the other nectin-1 molecule to form a homodimer, or to bind gD-mediating virus fusion. Differential binding modes for gD to HVEM and nectin-1 With the interaction interface in nectin-1 being primarily investigated, we then set out to explore those residues in HSV-1 gD potentially involved in nectin-1 binding. A total of 21 amino acids (including P23, L25, Q27, R36-H39, Q132, V214-F223, T230, V231 and Y234) were found to locate within 4.5Å distance from the nectin-1 entity ( Table 1 ). Of these residues, 7 locate within the N-terminal extension, 13 belong to the C-terminal extension and 1 is from the Ig core. Overall, these interface residues sterically congregate together to mainly form two surface patches ( Fig. 5a ). Patch 1 involves three residues at the distal N-terminus (P23, L25 and Q27) and three amino acids within the C-terminal α3-helix (T230, V231 and Y234), primarily contacting the FG-loop of the first Ig domain of nectin-1. Patch 2, on the other hand, with the remaining 15 residues, interacts in a much more extended manner with the nectin-1 [CC′C″FG] sheet. 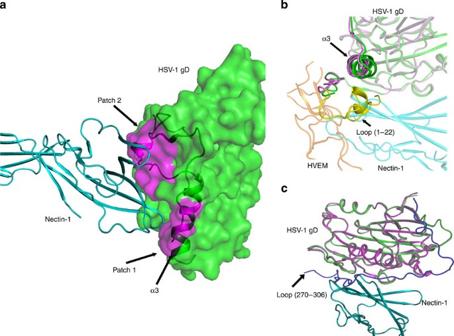Figure 5: Comparison of the binding modes between gD/nectin-1 and gD/HVEM. (a) The nectin-1 binding site within HSV-1 gD. Nectin-1 is presented as cyan ribbon. The gD molecule is shown in a surface representation. The interface residues sterically congregate together to mainly form two surface patches, which are highlighted in magenta colour and labelled. The terminal extensions and the α3-helix that were referred to in the text are indicated. (b) Superimposition of the complex structure of gD (green) binding to nectin-1 (cyan) onto that of gD (magenta) with HVEM (orange). The well-aligned gD molecules are indicated. The N-terminal 22 residues of gD (loop 1–22), which are absent in the gD/nectin-1 structure are coloured yellow and labelled. The α3-helix of gD is also highlighted. (c) Structural alignment of the gD/nectin-1 complex with a previously reported free gD of the entire ectodomain. The gD and nectin-1 molecules are coloured green and cyan, respectively, for the complex, whereas the free gD is shown in magenta. The C-terminal loop (270–306), which is only visible in the free gD structure, is highlighted in blue. Figure 5: Comparison of the binding modes between gD/nectin-1 and gD/HVEM. ( a ) The nectin-1 binding site within HSV-1 gD. Nectin-1 is presented as cyan ribbon. The gD molecule is shown in a surface representation. The interface residues sterically congregate together to mainly form two surface patches, which are highlighted in magenta colour and labelled. The terminal extensions and the α3-helix that were referred to in the text are indicated. ( b ) Superimposition of the complex structure of gD (green) binding to nectin-1 (cyan) onto that of gD (magenta) with HVEM (orange). The well-aligned gD molecules are indicated. The N-terminal 22 residues of gD (loop 1–22), which are absent in the gD/nectin-1 structure are coloured yellow and labelled. The α3-helix of gD is also highlighted. ( c ) Structural alignment of the gD/nectin-1 complex with a previously reported free gD of the entire ectodomain. The gD and nectin-1 molecules are coloured green and cyan, respectively, for the complex, whereas the free gD is shown in magenta. The C-terminal loop (270–306), which is only visible in the free gD structure, is highlighted in blue. Full size image It has long been believed that HSV-1 gD interacts with nectin-1 and HVEM in different manner [30] . To explore the molecular basis for the differential binding modes of gD to these two receptors, a previously solved structure of HSV-1 gD in complex with HVEM (PDB code: 1JMA) was selected for a comparison with our gD/nectin-1 structure. As shown in Figure 5b , superimposition of the two complex structures reveals a well-aligned gD molecule, with an RMSD of only 0.4 Å˚ for 209 Cα atoms. HVEM and nectin-1, however, bind to totally different steric parts of the gD protein. The major conformational differences in gD when bound to different receptors lie in the N-terminal 22 residues (loop 1–22) and the α3-helix. In the gD/HVEM complex, the loop (1–22) is part of a hairpin structure in which the HVEM binding site locates. The α3-helix, without a direct interaction with HVEM, is sandwiched between the hairpin and the barrel core. Nevertheless, in the gD/nectin-1 complex structure, the loop (1–22) is totally absent and α3-helix moves a small distance towards nectin-1 molecule. It should be noted that this distal loop covers the α3-helix and part of the N-terminal extension, which are of vital importance in nectin-1 binding. Therefore, binding of nectin-1 to gD will force the loop (1–22) to move away and simultaneously free the α3-helix, enabling a small shift to allow the C-terminal helix to interact with nectin-1. A previously reported free gD structure of the entire ectodomain (residues 1–306) [13] showed that the distal C-terminal residues were to extend, as a loop, to the vicinity of the N-terminal region. Superimposition of this structure (PDB code: 2C36) onto that of the gD/nectin-1 complex yields an RMSD of 0.307 ˚Å for 216 Cα pairs, demonstrating the conformational conservation for the main body of gD protein after nectin-1 binding. The long C-terminal loop (loops 270–306), as shown in Figure 5c , spreads over the gD/nectin-1 interaction interface. Therefore, nectin-1 binding should also displace the loop (270–306), which is believed to be involved in the activation of membrane fusion. Despite the different sites that HVEM and nectin-1 bind to, the two receptors share common features in the displacement of the gD C-terminus, implying a convergent fusion mechanism. This should also account for the previous observation that gD protein lacking the C-terminus exhibits much better binding capability than gD ectodomain of residues 1–306, as its binding to nectin-1 must involve moving gD C-terminus out of the way [13] , [25] . Hinge region plasticity between the nectin-1 Ig-like domains During our co-crystallization trials, we frequently obtained crystals of nectin-1 molecule alone from the complex preparations. One of these collected data sets, which is of 2.5 ˚Å in resolution, was also subjected to structural refinement. The final model, with R work =0.185 and R free =0.23, contains nectin-1 residues 36–335. Despite there being only one nectin-1 molecule per asymmetric unit, a single symmetry operation reveals a similar homodimer structure as observed in a recent report [21] . Structural alignment of this newly obtained nectin-1 structure (dubbed nectin-new) with the one in the gD/nectin-1 complex (dubbed nectin-com) and molecule A of the recently reported nectin-1 dimer structure (dubbed nectin-homo) reveals well-aligned first and second Ig-like domains, but relatively discrepant domain 3 ( Fig. 6a ). The major difference lies in the interdomain angles between domains 2 and 3. With the longitudinal axis crossing the first two domains of nectin-1 as reference, the orientation of the third Ig-like domain within the three nectin-1 structures solved could be quantitatively compared. 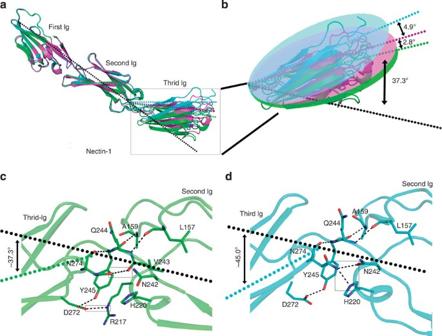Figure 6: Comparative analysis of the hinge region between the second and third Ig-like domains of the nectin-1 in different crystallization conditions. (a) A superimposition overview of the three nectin-1 structures referred to in the text. The two structures of free and bounded forms solved in this study (dubbed nectin-new and nectin-com, respectively), and molecule A of an earlier reported homodimer structure (dubbed nectin-homo) are aligned and coloured green, magenta and cyan, respectively. The well-aligned first and second Ig-like domains are presented, with a black dashed line indicating the longitudinal axis crossing these two domains. The third Ig-like domain, which exhibited obvious orientation differences, is highlighted by marking with a black box. The coloured dash lines represent respective orientations of the third domain within the three nectin-1 structures. (b) A magnified view of the third Ig-like domains presented in (a). The interdomain angle differences in the three nectin-1 structures are labelled and their relative positions are eclipsed. (c,d) Detailed interdomain interactions between the second and third Ig-like domains of nectin-1. Those residues referred to in the text are shown in a stick representation and labelled. Slim dashed lines indicated H-bond or salt-bridge interactions. Those H-bond differences between nectin-new and nectin-homo are highlighted by marking with black boxes. (c) Nectin-new. (d) Nectin-homo. As shown in Figure 6b , nectin-homo exhibits the least extended conformation, showing an interdomain angle of about 45.0°, followed by nectin-com with an angle of about 40.1°. The one closest to a rod-shape is nectin-new, whose domain 3 forms an angle of only 37.3° with domain 2. These observations indicate a rigid hinge between the first and second domains, but a relatively flexible interdomain linker for the second and third Ig-like domains. Figure 6: Comparative analysis of the hinge region between the second and third Ig-like domains of the nectin-1 in different crystallization conditions. ( a ) A superimposition overview of the three nectin-1 structures referred to in the text. The two structures of free and bounded forms solved in this study (dubbed nectin-new and nectin-com, respectively), and molecule A of an earlier reported homodimer structure (dubbed nectin-homo) are aligned and coloured green, magenta and cyan, respectively. The well-aligned first and second Ig-like domains are presented, with a black dashed line indicating the longitudinal axis crossing these two domains. The third Ig-like domain, which exhibited obvious orientation differences, is highlighted by marking with a black box. The coloured dash lines represent respective orientations of the third domain within the three nectin-1 structures. ( b ) A magnified view of the third Ig-like domains presented in ( a ). The interdomain angle differences in the three nectin-1 structures are labelled and their relative positions are eclipsed. ( c , d ) Detailed interdomain interactions between the second and third Ig-like domains of nectin-1. Those residues referred to in the text are shown in a stick representation and labelled. Slim dashed lines indicated H-bond or salt-bridge interactions. Those H-bond differences between nectin-new and nectin-homo are highlighted by marking with black boxes. ( c ) Nectin-new. ( d ) Nectin-homo. Full size image We then analysed in detail the interdomain interactions between the second and the third Ig-like domains within nectin-new and nectin-homo, which are the two structures exhibiting the biggest angle difference. As shown in Figure 6c,d , in both structures, the interdomain-stabilizing network involves six strong polar interactions (H-bond or salt-bridge). Four H-bonds were shared by both nectin-new and nectin-homo, including the main-chain hydrogen bonds within A259/Q244, L157/Q244 and Y245/N274, as well as a side-chain H-bond formed between Y245 and D272. Nectin-new contains an additional hydrogen bond between V243 and N274, and a salt-bridge within the side-chains of D272 and R217. Nevertheless, within nectin-homo, two extra H-bond interactions were observed to form among the side-chains of H220, N242 and N274. It should be noted that residues H220 and N242 are relatively farther away from the third domain than residues V243 and R217. We believe the two H-bonds conferred by H220 and N242 will cause the nectin-1 third domain to bend further, leading to an increased interdomain angle between the second and the third Ig-like domains. Furthermore, in both nectin-new and nectin-homo, equal amounts of stabilizing bonds were formed, indicating that either conformation could be energetically preferable. Therefore, with an overall rod-shape remaining unchanged, the rigid nectin-1 molecule still exhibits limited flexibility by changing between a relatively extended conformation (as represented by nectin-new) and a relatively bent conformation (as represented by nectin-homo). Owing to limited diffraction resolution, we are unable to define the inter-domain (between the second and the third Igs) H-bonds or salt-bridges for the nectin-1 (nectin-com) in the gD/nectin-1 complex; however, with different angles present we would expect to see a distinct interaction in addition to the main conserved interaction. Many pathogens, including viruses, use host factors (proteins) to exert their survival strategy and exploit the host normal functions. In this manner the virus escapes from the immune surveillance and in some cases, like HSV, persists into latency. In addition to its initial role in virus initial entry, it has been shown that binding of the HSV-1 surface envelope protein gD to CAMs molecule nectin-1 in infected cells would assist the virus to spread to uninfected cells [24] , [28] , [31] . Herein, through complex crystallography, the binding mode of HSV-1 gD with its second receptor nectin-1 is clearly unveiled for the first time. The 1:1 binding mode makes the nectin-1 dimerization impossible and precludes the nectin-1-mediated cell–cell adhesion. This observation is consistent with the previous functional studies showing that monoclonal antibody mapping onto the first IgV domain of nectin-1 could block gD binding, and soluble gD and HSV-1 are both able to prevent nectin-1-mediated cell aggregation [23] , [28] . It is also notable that recent crystallography work on nectin-1 cis -dimer and previous functional work would speculate a 2:1 (2 nectin-1:1 gD) or a 2:2 (2 nectin-1:2 gD) model [21] , [22] . In these models, the nectin-1 dimerization is also a prerequisite for the gD binding. Our results reported here clearly rule this out. Of course in the in vivo situation, the circumstances within the virus/host interface could be much more complicated. With the interaction mode of gD with nectin-1 being illustrated at the atomic level in this study, further investigations are needed to dissect the detailed entry mechanism of HSV, including the difference between HSV-1 and HSV-2, if there is any. In addition, calcium is also a key factor involved in HSV entry. Although nectin-1 itself is a calcium-independent CAM molecule, previous studies have shown that depletion of the metal could cause the disruption of the adherens junctions in which nectin-1 accumulate. The herein exposed nectin-1 molecule should be more accessible to virus gD as the complex structure reported here demonstrate that nectin-1/gD interaction requires the dissociation of nectin-1 dimer, if the dimer is the physiological form [32] . The observed nectin-1/gD binding mode might also indicate a possibility that gD could mimic natural nectin-1 in trans interaction to prevent potentially adverse or to promote potentially beneficial cellular signalling for virus infection. Despite that the nectin-1-mediated signalling pathway remains largely unknown, a previous study indeed shows an increase of the intracellular calcium level during HSV infection [33] . This change in calcium concentration requires the nectin-1/gD interaction, and could in turn facilitate virus entry [34] . Further work is needed to investigate the cellular signalling pathway response to the binding of gD to nectin-1. Structural and biophysical data in this study also demonstrate that nectin-1 exists in solution, possibly on the cell surface as well, as a monomer–dimer equilibrium as has been illustrated in a recent publication [21] . In our effort to obtain the complex crystals, we kept getting nectin-1 alone crystals from time to time out of the protein mixture. Finally we managed to obtain a diffraction-quality crystal for the complex when the nectin-1 monomer peak was carefully selected. This result further confirms the 1:1 binding mode, and moreover the nectin-1 dimer would not bind to gD. Therefore, we speculate that there is only one homodimeric binding format for nectin-1 and interaction of both the cis -homodimer and trans -dimer is the same. Narita et al . [21] argued in their model of differential dimer formats for cis -homodimer and trans -homodimer of nectin-1 that the perpendicular interaction (almost 90° between the two molecules) of nectin-1 dimer can only assist cis -interaction (on the same cell surface) because there is not enough angles for two cells to interact in their trans -dimer. This notion is indirectly supported by a dimeric structure of Necl-1 in that the two molecules formed a more open angle (approximately 110°) [35] , which is believed to represent a trans -dimer of the family. The two crystal structures (free and complex) of the three Ig domains of nectin-1 in our study and the earlier reported structure [21] show that the hinge region between the second Ig-like domain and the third Ig-like domain of nectin-1 has some flexibility, unlike the hinge between the domains 1 and 2. Flexible hinge regions for Ig molecules are not uncommon [36] . We propose here that this flexibility would overcome the angle problem for the cell interaction in the trans -dimer and the dimer form we found here represents both the cis - and trans -dimer of the nectin-1. It is also noteworthy that there are 32 amino acids between the third Ig domain and the transmembrane domain in nectin-1, which could allow for more flexibility. Although our explanation for the binding interface between gD and nectin-1 has some limitations due to low resolution (3.2 ˚Å) the complex structure solved here fundamentally confirms the assumptions from the previous mutational work [30] , [37] , [38] , [39] , [40] , [41] . Using 4.5 ˚Å as a cutoff point (van der Waals force and above) from our complex structure, 21 amino acids from gD are involved in the gD/nectin-1 complex interaction, 7 of them from the N-terminal extension, 13 from the C-terminal extension and 1 from the Ig core. In consistence with our finding, Y38 was found to be essential for both binding to nectin-1 and cell fusion and both R36A and H39A mutations impaired the binding to Nectin-1 (ref. 42 ). Some inconsistent results were reported from different laboratories [38] , [42] as to other amino acids of gD in nectin-1 binding, including the only potential amino acid, Q132, in the Ig core [42] . Although about 22 amino acids in nectin-1 are involved in its interaction with gD (4.5 ˚Å cutoff) from our complex structure, previous limited mutational work only identified three residues involved: Q76, N77 and M85 (refs 27 , 43 ). Therefore, our complex structure clearly defines the distinctive nectin-1 binding mode to gD, and will assist in our understanding of HSV fusion. Binding modes of gD to HVEM and nectin-1 are totally different. However, owing to the N-terminal extension involvement in both binding modes (some common interacting amino acids, for example, L25 and Q27, are involved in both cases), it is impossible for gD to bind the two receptors simultaneously. Consistent with our structure, earlier work shows that soluble nectin-1 blocks virus entry into HVEM-expressing CHO cells and in turn HVEM impairs the virus entry into nectin-1-expressing cells [44] . The tissue expression patterns support the alternate receptor functions as nectin-1 is mainly expressed in epithelial, neuronal, endothelial cells and keratinocytes [45] , but HVEM has a more wide-spectrum of tissue expressions, including T lymphocytes and trabecular meshwork cells, as well as lung, liver, kidney and lymphoid tissues [46] , [47] . Therefore, the two receptors are used by HSV-1 as its alternate entry/fusion mediators, depending on the infected tissues. As the binding modes of gD to nectin-1 is almost the same as nectin-1 dimer interaction, the effect of gD binding to nectin-1 on the host cells, that is, on the HSV-1 pathogenesis, should be further studied. Despite different modes of HSV-1 gD binding to HVEM and nectin-1, we provide solid structural evidence that the two receptors share a common feature in terms of gD C-terminus displacement. It is widely accepted that the C-terminus of gD has a pivotal role in activating the viral/host membrane fusion and is thereby also proposed as a profusogenic domain (PFD) [5] , [14] . However, the exact mechanism on PFD-mediated fusion activation remains a mystery. One hypothesis favours a prelocated PFD in the receptor-binding site of gD 13 , and gD/receptor interactions could result in a displacement of the PFD, enabling its exposure to the fusogenic glycoproteins B, H and L. The complex structure reported in this study seems to favour this viewpoint as binding of nectin-1 to gD indeed will cause a relocation of the gD C-terminus, especially the PFD. Whereas other studies show that chimeric gDs using uPA or IL13, or the HER2 antibody, to substitute the N-terminal domain of gD, are all functionally active in mediating virus entry into cells expressing the respective cognate receptors [41] , [48] , [49] . Although it cannot be completely ruled out, it is unlikely that three irrelevant ligands (uPA, IL13 and HER2 antibody) could cause identical conformational changes in the PFD. Without direct evidence, an interaction of gD with the core fusion machinery that is independent of the conformational changes in gD PFD could not be excluded. Further structural and functional studies are needed to settle these issues. In conclusion, the solution of the gD and nectin-1 complex structure clearly depicts a picture for the receptor-viral envelope protein interaction mode and the differential functions of nectin-1 dimer and monomer. Moreover, this discovery opens up new opportunities for structure-based fusion-inhibitor design for HSV-1. Preparation of soluble proteins The ectodomain covering three Ig-like domains of the human nectin-1 (amino acids 30–335) was cloned into an E. coli expression system (pET21b, Invitrogen) following the reported methods [21] . The protein was expressed as inclusion bodies and the inclusion bodies were prepared in the buffer of 100 mM Tris, pH 9.0, 400 mM L -arginine, 2 mM EDTA, 4 M urea, 5 mM reduced glutathione and 1 mM oxidized glutathione. For refolding, the inclusion bodies were first dialysed against water for 8 h and then against a buffer of 10 mM Tris, pH 9.0, 10 mM NaCl, for another 8 h. The samples were then subjected to a gel-filtration on a Hiload 16/60 Superdex 200 column (GE Healthcare). Usually a few peaks could be seen and estimation of their M W s would correlate to oligomer, dimer and monomer. If the protein concentration is well controlled, monomer/dimer peaks could be obtained. HSV-1 (KOS strain) gD ectodomain of residues 1 to 285 (gD285) was expressed by using the Bac-to-Bac baculovirus expression system (Invitrogen). The cDNA fragment covering amino acids 1–285 was cloned into pFastBac vector with a C-terminal 6-his tag. The vector had been previously modified to incorporate the baculovirus gp67 signal sequence [50] , [51] , [52] . The recombinant baculovirus was used to infect Hi5 cells for the production of the soluble gD. The proteins were purified from the Hi5 cell supernatants first by nickel affinity chromatography (GE Healthcare) and then gel-filtration chromatography using a Superdex 200 column (GE Healthcare) for further purification. Biochemical/biophysical characterizations of the proteins Gel-filtration analysis for the M W estimation was performed by using a Superdex 200 column (10/300 GL) with purified proteins. Separately purified gD and nectin-1 was mixed in a ratio of 1:1 and the mixture was incubated on ice for 4 h, after which it was loaded onto the column. At the same time the purified gD or nectin-1 was run onto the same column and the chromatographs were superimposed for M W comparison. Analytical ultracentrifugation was performed on a Beckman XL-A analytical ultracentrifuge. The nectin-1 sample was used at an initial concentration of A 280 =0.8 absorbance units and dissolved in 20 mM Tris-Cl, 150 mM NaCl, pH 9.0. Samples (400 μl) and reference solutions (400 μl, 20 mM Tris-Cl, 150 mM NaCl, pH 9.0) were loaded into a conventional double-sector quartz cell and mounted in a Beckman Coulter An-60 Ti 4-hole rotor. Sedimentation velocity experiments were performed at a speed of 60,000 r.p.m. The protein profiles were measured by ultraviolet absorbance at 280 nm in a continuous mode with time intervals of 480 s. The recorded scans for the various time points were collected and analysed using the c(s) continuous size distribution model with the SEDFIT programme Version 11.3b. Molecular weights were estimated using the c(M) model after fitting the frictional ratio ( f/f0 ). SPR measurements The binding kinetics between the soluble gD and nectin-1 was analysed at 25 °C on a BIAcore 3000 machine with CM5 chips (GE Healthcare). HBS-EP buffer (10 mM HEPES, 150 mM NaCl, 3 mM EDTA, 0.005% Tween 20) was used for all measurements. For SPR measurements, both gD and nectin-1 were purified by gel filtration using Superdex 200 column (GE Healthcare). We used the blank channel as negative control. About 1,000 response units of nectin-1 were immobilized on the chip, followed by blockade with EDTA. When the data collection was finished in each cycle, the sensor surface was regenerated with 10 mM NaOH. A serial of concentrations ranging from 1 to 0.0156 μM were designed for the experiment. Sensograms were fit globally with BIAcore 3000 analysis software (BIAevaluation Version 4.1) using 1:1 Langumuir binding mode. Crystallization gD/nectin-1 complex crystals or nectin-1 alone crystals were grown using the hanging-drop vapour diffusion method. Two methods were used for gD/nectin-1 complex crystallization trials. First, two proteins were separately purified by gel-filtration chromatography and mixed in a 1:1 ratio. The mixture was further purified by gel-filtration chromatography using a Superdex 200 column (GE Healthcare) and the complex peak was carefully collected. The second method was to mix the separately purified gD and nectin-1 in a 3:1 molar ratio and directly to set up the crystallization trials without further purification. Initial screening was performed using a commercial kit (Hampton Research). Diffraction quality crystals were obtained by mixing 1 μl of the concentrated protein at 4 mg ml −1 in 20 mM Tris, pH 7.5, and 50 mM NaCl with 1 μl of the kit-screening buffer. For the first diffraction-quality crystal, 20% PEG 2,000, 0.2 M trimethylamine N -oxidedihydrate, 0.1 M Tris, pH 8.5, was used (crystal growing temperature was 16 °C) and the crystal turned out to be nectin-1 homodimer alone, although the complex protein mixture was used. gD/nectin-1 complex crystal grew at 4 °C in the buffer of 20% PEG 1,000, 0.1 M lithium sulphate monohydrate, 0.1 M sodium citrate tribasic dehydrate, pH 5.5, by using the second method. Data collection and processing, and structure solution Nectin-1/gD complex and nectin-1 crystals were first incubated in mother liquor containing 20% of glycerol, and then flash-cooled at 100 K. Diffraction data were collected at SSRF beamline BL17U. Diffraction data were processed and scaled using HKL2000 (ref. 53 ). Data collection and processing statistics are summarized in Table 2 . Both the structures of nectin-1 and nectin-1/gD complex were solved by molecular replacement method using Phaser [54] from the CCP4 programme suite [55] with the structure of Nectin-1 (PDB code: 3ALP) and HSV-1 gD (PDB code: 1L2G) as the search models. Initial restrained rigid-body refinement and manual model building were performed by using REFMAC5 (ref. 56 ) and COOT [57] , respectively. Further rounds of refinement were performed using the phenix.refine programme implemented in the PHENIX package [58] with rigid-body refinement, isotropic ADP refinement and TLS refinement. The stereochemical quality of the final model was assessed with the programme PROCHECK [59] . 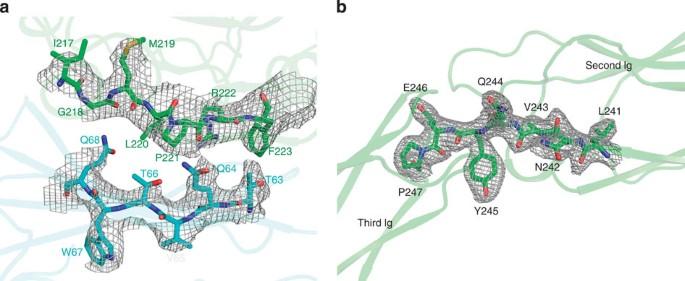Figure 7: Representative electron densities for both the complex and the free nectin-1 structures solved in this study. The densities were generated by contour at 1.0σ using a 2|Fo|-|Fc|map. (a) Part of the gD/nectin-1 interface. Seven residues from HSV-1 gD (I217–F223) and six amino acids of nectin-1 (T63–Q68) are shown in stick representation, and coloured green and cyan, respectively. (b) A seven-residue linker connecting the second and the third Ig-like domains of nectin-1 within the structure of nectin-new. The residues involved are shown in stick and labelled. Overall electron densities of both the complex and the free nectin-1 molecule are shown in Figure 7 . The Ramachandran plot distribution for the residues in the gD/nectin-1 complex structure was 88.8, 10.1, and 1.1% for the most favored, additionally and generously allowed regions, respectively. These values were 88.5, 10.3, and 1.1% for the nectin-1 structure. The figures were generated using PyMOL ( http://pymol.sourceforge.net ). The atomic coordinates and structure factors of the structures solved in this study have been deposited into the Protein Data Bank ( Table 2 ). Table 2 Data collection and refinement statistics. Full size table Figure 7: Representative electron densities for both the complex and the free nectin-1 structures solved in this study. The densities were generated by contour at 1.0σ using a 2|Fo|-|Fc|map. ( a ) Part of the gD/nectin-1 interface. Seven residues from HSV-1 gD (I217–F223) and six amino acids of nectin-1 (T63–Q68) are shown in stick representation, and coloured green and cyan, respectively. ( b ) A seven-residue linker connecting the second and the third Ig-like domains of nectin-1 within the structure of nectin-new. The residues involved are shown in stick and labelled. Full size image Accession codes: Atomic coordinates and structure factors for gD/nectin-1 and nectin-1 alone have been deposited in the Protein Data Bank under the accession codes 3U82 and 3U83 . How to cite this article: Zhang, N. et al . Binding of herpes simplex virus glycoprotein D to nectin-1 exploits host cell adhesion. Nat. Commun. 2:577 doi: 10.1038/ncomms1571 (2011).